Genome-wide association study identifies 14 novel risk alleles associated with basal cell carcinoma Basal cell carcinoma (BCC) is the most common cancer worldwide with an annual incidence of 2.8 million cases in the United States alone. Previous studies have demonstrated an association between 21 distinct genetic loci and BCC risk. Here, we report the results of a two-stage genome-wide association study of BCC, totalling 17,187 cases and 287,054 controls. We confirm 17 previously reported loci and identify 14 new susceptibility loci reaching genome-wide significance ( P <5 × 10 −8 , logistic regression). These newly associated SNPs lie within predicted keratinocyte regulatory elements and in expression quantitative trait loci; furthermore, we identify candidate genes and non-coding RNAs involved in telomere maintenance, immune regulation and tumour progression, providing deeper insight into the pathogenesis of BCC. With 2.8 million new cases diagnosed annually in the United States [1] , basal cell carcinoma (BCC) is the most common cancer worldwide and contributes substantially to morbidity. BCC risk has been associated with ultraviolet (UV) exposure, fair skin, arsenic exposure, ionizing radiation, chronic immunosuppression, male gender and age [1] . Since 2008, six population-based genome-wide association studies (GWAS) of BCC have been reported identifying 16 regions of susceptibility [2] , [3] , [4] , [5] , [6] , [7] . Candidate gene studies have identified five additional pigmentation loci associated with BCC, including IRF4 , SLC45A2 , RALY , TYR and OCA2 [7] . Here, we report the largest-to-date two-stage genome-wide association meta-analysis for BCC totalling 17,187 cases and 287,054 controls. The results of this study confirm 12 of 16 loci from prior GWAS, along with 5 of 5 loci from previous candidate gene studies, and identify 14 novel susceptibility loci for BCC. 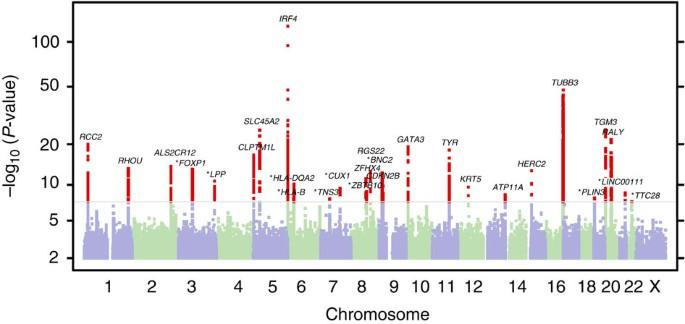Figure 1: Manhattan plot of stage 1 GWAS analysis of BCC from 23andMe data set. Total stage 1 GWAS analysis included 12,945 cases and 274,252 controls. Loci with smallestP<10−6(28 total, logistic regression) are labelled with the name of the nearest gene. Positions withP<5 × 10−8(genome-wide significance) are shown in red. In stage 1, ten novel BCC susceptibility loci reached genome-wide significance after adjusting for genomic control, all of which are labelled in the figure with asterisks: from left to right,3p13(FOXP1),3q28(LPP),6p21.32(HLA-DQA2),6p21.33(HLA-B),7p12.3(TNS3),7q22.1(CUX1),8q21.13(ZBTB10),9p22.2(nearBNC2),19p13.3(PLIN3),21q22.3(LINC00111). Four additional novel susceptibility loci—6p21.3(NEU1),10q24.3(OBFC1),6q27(MIR3939),6p22.3(CASC15)—were genome-wide significant in the overall meta-analysis (Table 2) and thus are not labelled in the figure. Stage 1 consisted of 12,945 self-reported BCC cases and 274,252 controls of European ancestry from 23andMe research participants ( Supplementary Table 1 ). 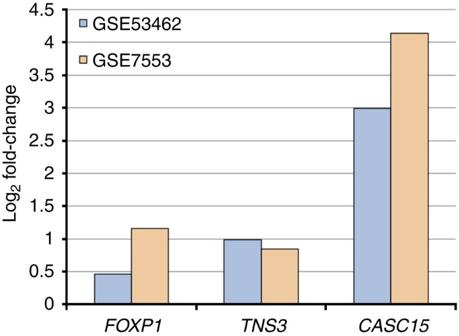Figure 2: Gene expression analysis for novel BCC susceptibility loci. Processed microarray expression data were obtained from Gene Expression Omnibus (GSE53462, blue, and GSE7553, orange). Transcript levels in BCC samples were compared to levels in normal skin controls via Geo2R. Three genes—FOXP1,TNS3andCASC15—were significantly upregulated in BCC relative to normal skin (P<0.05, linear models for microarray analysis) in both data sets. Validation of self-reported surveys with adjudicated medical records revealed a sensitivity and specificity of 93% and 99%, respectively ( Supplementary Table 2 ), indicating a misclassification rate of less than 10%. Simulation analysis demonstrated that this misclassification rate only modestly reduced the power to detect associations in this study ( Supplementary Fig. 1 ). Stage 2 consisted of an independent GWAS cohort of 4,242 BCC cases and 12,802 controls of European ancestry from the Nurses’ Health Study and Health Professionals Follow-Up Study ( Supplementary Table 1 ). Subsequently, meta-analysis of stages 1 and 2 was performed, encompassing 17,187 cases and 287,054 controls ( Supplementary Table 1 ). Further information on methodology and imputation quality control is presented in the Online Methods, Supplementary Tables 3-5 , and Supplementary Figs 2–7 . Stage 1 analysis Twenty-eight index single nucleotide polymorphisms (SNPs) were associated with BCC at the genome-wide significance level ( P <5.0 × 10 −8 , logistic regression) in stage 1 and are depicted in the Manhattan plot ( Fig. 1 ). Subset analysis revealed relatively consistent effect sizes across age and gender for these 28 SNPs ( Supplementary Tables 6–7 , Supplementary Fig. 8 ). Interestingly, slightly larger effect sizes tended to occur in younger cases, suggesting that other risk factors may play an increasing role with age. As 10% of the BCC cases in our stage 1 cohort subsequently developed melanoma, we also investigated whether the co-occurrence of melanoma contributed to the observed associations with BCC risk. We therefore computed association tests for the stage 1 index SNPs in BCC cases with and without melanoma. All 28 SNPs displayed consistent effect sizes across the two groups ( Table 1 , Supplementary Fig. 9 ), indicating that they are independently associated with BCC susceptibility. Figure 1: Manhattan plot of stage 1 GWAS analysis of BCC from 23andMe data set. Total stage 1 GWAS analysis included 12,945 cases and 274,252 controls. Loci with smallest P <10 −6 (28 total, logistic regression) are labelled with the name of the nearest gene. Positions with P <5 × 10 −8 (genome-wide significance) are shown in red. In stage 1, ten novel BCC susceptibility loci reached genome-wide significance after adjusting for genomic control, all of which are labelled in the figure with asterisks: from left to right, 3p13 ( FOXP1 ), 3q28 ( LPP ), 6p21.32 ( HLA-DQA2 ), 6p21.33 ( HLA-B ), 7p12.3 (TNS3 ), 7q22.1 ( CUX1 ), 8q21.13 ( ZBTB10 ), 9p22.2 (near BNC2 ), 19p13.3 ( PLIN3 ), 21q22.3 ( LINC00111 ). Four additional novel susceptibility loci— 6p21.3 ( NEU1 ), 10q24.3 ( OBFC1 ), 6q27 ( MIR3939 ), 6p22.3 ( CASC15 )—were genome-wide significant in the overall meta-analysis ( Table 2 ) and thus are not labelled in the figure. Full size image Table 1 Interaction of 28 genome-wide significant BCC associations in stage 1 with melanoma. Full size table Stage 2 and combined meta-analysis Twenty of the 28 index SNPs were replicated in the stage 2 analysis ( P <0.05, logistic regression). While some loci did not reach statistical significance in stage 2, their 95% confidence intervals (for odds ratios) overlapped with the corresponding stage 1 confidence intervals. Meta-analysis of stages 1 and 2 identified a total of 31 loci reaching genome-wide significance ( P <5 × 10 −8 , logistic regression) for association with BCC. Among these 31 loci, 17 are previously reported ( Supplementary Tables 8–12 ). The remaining 14 are novel BCC susceptibility loci ( Table 2 , Supplementary Table 13 ). Forest plots and regional association plots for these 14 SNPs are provided in Supplementary Figs 10–12 . Of these 14 novel risk variants, 10 reached genome-wide significance in stage 1 and 4 reached genome-wide significance in the combined meta-analysis. As many pigmentation loci have been associated with BCC susceptibility, we adjusted for pigmentation phenotype in our stage 2 cohort and did not observe a significant difference between adjusted and unadjusted results for the 14 novel risk variants ( Supplementary Table 14 ). Table 2 Fourteen novel loci reaching genome-wide significance in two-stage GWAS of BCC. Full size table Heritability of BCC and gene expression analysis To measure the proportion of BCC heritability that can be attributed to these SNPs, we calculated the familial relative risk for BCC as outlined by the Cancer Oncological Gene-Environment Study. Overall, 10.98% of familial relative risk for BCC is explained by the 31 genome-wide significant loci; of this percentage, the 14 novel susceptibility loci account for 2.62%. To further explore the role of these 14 loci in BCC pathogenesis, we evaluated expression levels of nearby genes in BCC tissue using two data sets from the Gene Expression Omnibus (GEO) (GSE53462 and GSE7553). Three loci demonstrated significant differential gene expression in BCC relative to normal skin: 3p13 FOXP1 , 7p12.3 TNS3 and 6p22.3 CASC15 ( Fig. 2 , P <0.05, linear models for microarray analysis). Figure 2: Gene expression analysis for novel BCC susceptibility loci. Processed microarray expression data were obtained from Gene Expression Omnibus (GSE53462, blue, and GSE7553, orange). Transcript levels in BCC samples were compared to levels in normal skin controls via Geo2R. Three genes— FOXP1 , TNS3 and CASC15 —were significantly upregulated in BCC relative to normal skin ( P <0.05, linear models for microarray analysis) in both data sets. Full size image Gene-environment interaction analysis Ultraviolet exposure and pigmentation phenotypes have been associated with BCC risk and may interact with genetic variants to confer BCC susceptibility. To further explore the influence of such factors on our study, we tested for interactions between all 31 significant loci and UV exposure, hair colour, number of sunburns and tanning ability ( Supplementary Table 15 ). This analysis revealed only one significant interaction, between rs191177147 ( LPP ) and hair colour. Additional testing in three separate hair colour groups demonstrated that rs191177147 significantly interacted with the light brown and dark brown/black hair groups ( Table 3 , P =2.9 × 10 −6 , logistic regression). Table 3 Stage 2 subset analysis of novel BCC risk variant rs191177147 (3q28, LPP ) in different hair colour subgroups. Full size table The 14 novel susceptibility loci cluster into five functional categories: telomere biology, immune regulation, tumour progression, non-coding RNA and pigmentation. Variants within the TERT locus have previously been associated with BCC susceptibility, thus implicating telomere regulation in BCC development [8] . Here, we identify a novel BCC susceptibility locus, OBFC1 , that is also involved in telomere maintenance. rs7907606 at 10q24.3 ( P =4.7 × 10 −9 , odds ratio (OR)=1.10, logistic regression) lies 3 kb upstream of the OBFC1 gene, a member of the heterotrimer CST complex [8] . This complex restricts telomere extension by binding telomeric DNA and disrupting the ability of other proteins to recruit telomerase [9] . Variants in the OBFC1 locus have been associated with mean leukocyte telomere length [8] , [10] . rs7907606 is in linkage disequilibrium (LD) with four of these variants ( Supplementary Table 16 ), including rs4387287 ( r 2 =0.98, D ′=−1.00), which lies within the promoter of OBFC1 and is an eQTL for this gene in sun-exposed skin ( P =8.3 × 10 −6 , GTEx V6 analysis) [11] . Though widely studied, the connection between telomere length and cancer is context dependent, as both long and short telomeres are linked to malignancy [12] . This discrepancy is readily apparent in the context of skin cancer, where longer telomeres are associated with melanoma and shorter telomeres are associated with BCC [12] . Our results further implicate telomere homeostasis in BCC pathogenesis. We also identified six novel susceptibility loci associated with immune regulation. Two SNPs, rs1050529 and rs9275642, are in human leukocyte antigen (HLA) regions. rs1050529 at 6p21.33 ( P =2.6 × 10 −9 , OR=0.90, logistic regression) lies within an exon of HLA-B , and leads to a non-conservative amino acid substitution (A65T). rs1050529 has predicted enhancer and promoter activity in keratinocytes and is an eQTL in six tissues. Variants in HLA-B have been associated with a range of autoimmune conditions, including vitiligo and psoriasis [13] , [14] . HLA-B encodes the heavy chain component of major histocompatibility complex (MHC) class I molecules, which present endogenously synthesized peptides to cytotoxic T cells. Downregulation of MHC class I molecules is a feature of many types of cancers, which is thought to enable tumour cells to evade recognition and destruction by T cells [15] . An analysis of 91 human melanoma cell lines revealed decreased expression of class I molecules in 67% of the cell lines, with HLA-B being the most common [16] . The second HLA SNP reaching genome-wide significance was rs9275642 at 6p21.32 ( P =2.4 × 10 −12 , OR=0.89, logistic regression), which is located 24 kb upstream of HLA-DQA2 . This SNP is in tight LD with rs9275640 ( r 2 =0.89, D′=0.99), which is an eQTL for this gene in sun-exposed skin ( P =3.6 × 10 −6 , GTEx V6 analysis) [11] . HLA-DQA2 variants are also associated with autoimmune diseases, including type 1 diabetes, rheumatoid arthritis and alopecia areata [14] . These findings represent the first genome-wide significant association between MHC genes and BCC risk. The third immune-related SNP, rs191177147 at 3q28 ( P= 9.8 × 10 −17 , OR=1.11, logistic regression), resides within an intron of LPP and is in LD with rs1464510 ( r 2 =0.54) and rs9860547 ( r 2 =0.68, Supplementary Table 17 ); the former is associated with autoimmune diseases such as celiac disease, rheumatoid arthritis, juvenile idiopathic arthritis and vitiligo [17] , [18] , [19] , while the latter is associated with allergy [20] . LPP encodes an intracellular protein that shuttles between the cell membrane and the nucleus, where it interacts with transcription factors to modulate gene expression [21] . LPP overexpression has been reported in squamous cell lung carcinomas and primary sarcomas [21] . We also found an association between rs191177147 and hair colour, suggesting that this SNP may also contribute to BCC risk by altering pigmentation phenotypes. Another SNP with potential significance in immune regulation is rs10425559 at 19p13.3 ( P= 2.9 × 10 −9 , OR=0.93, logistic regression), which is intergenic and flanked by TICAM1 and PLIN3 . It is linked to rs7255265 ( r 2 =0.68, D ′=0.9, Supplementary Table 18 ), which is located in an exon of TICAM1 and has predicted enhancer activity in keratinocytes. TICAM1 is an intracellular toll-like receptor(TLR) adaptor molecule involved in innate immunity; moreover, it acts as a pro-apoptotic tumour suppressor by mediating the interaction between TLR-3 and caspase-8 in some malignancies, including melanoma [22] . PLIN3 encodes a cytosolic protein that binds to the GTPase RAB9, a member of the RAS oncogene family [23] . Overexpression of PLIN3 has been linked to cervical carcinoma [24] . The fifth immune-related SNP, rs9267650 at 6p21.3 ( P= 1.1 × 10 −8 , OR=1.17, logistic regression), lies 0.5 kb downstream of NEU1 , which encodes a lysosomal enzyme implicated in many diverse processes, including activation of TLRs [25] , wound healing [26] , [27] and suppression of ovarian carcinoma [28] . Finally, rs11993814 at 8q21.13 ( P =1.1 × 10 −12 , OR=0.91, logistic regression), located 9 kb upstream of ZBTB10 , is an eQTL in two tissues and is in LD with rs6998967 ( r 2 =0.6, D ′=1.0), associated with late-onset myasthenia gravis [29] . ZBTB10 encodes a zinc finger transcription factor involved in regulating the expression of Interleukin-10 through suppression of Sp1 [29] , [30] , [31] . Abnormal interaction between ZBTB10 and Sp1 is seen in several different cancer cell lines, with ZBTB10 consistently exhibiting tumour-suppressing activity [32] . All together, these findings implicate a number of immune regulatory loci in BCC susceptibility. Four of our novel susceptibility loci are associated with tumour progression. rs2116709 at 3p13 ( P= 5.7 × 10 −16 , OR=0.91, logistic regression) resides within an intron of FOXP1 , a transcription factor that, in addition to regulating organ development, acts as a tumour suppressor in some cancers (for example, prostate [33] ) and as an oncoprotein in others (for example, oesophagus [34] ). It is overexpressed in oesophageal cancer and many types of lymphomas, including cutaneous B-cell lymphomas [34] , [35] . Similarly, we found that FOXP1 is significantly overexpressed in BCC as compared with normal skin controls. Our findings suggest a role for FOXP1 in BCC development. rs73183643 at 7q22.1 ( P= 1.3 × 10 −13 , OR=0.91, logistic regression) is located 40 kb upstream of CUX1 , which encodes a homeodomain-containing transcription factor involved in cell proliferation and differentiation. Both in vitro and in vivo studies have shown that CUX1 promotes tumorigenesis in a range of neoplasms, including melanoma and pancreatic cancer, by increasing cell motility and inhibiting apoptosis [36] , [37] . Another tumorigenesis-related SNP, rs7776701 at 7p12.3 ( P= 2.0 × 10 −8 , OR=0.94, logistic regression), lies within an intron of TNS3 and has enhancer activity in 14 tissues, including keratinocytes. This SNP is in LD with rs56232506 ( r 2 =0.76, D ′=0.99), also intronic to TNS3 and associated with prostate cancer [38] . Tensin-3, the cytosolic protein product of TNS3 , connects transmembrane proteins to cytoskeletal elements and influences cell migration [39] . Studies of human metastatic melanoma, non-small cell lung cancer and breast cancer cell lines demonstrate that reduced expression of TNS3 corresponds to dramatic inhibition of cell proliferation and migration, suggesting that TNS3 is an oncogene [39] . This idea is consistent with our expression analysis, in which TNS3 was significantly upregulated in BCC. The fourth SNP in this category, rs4710154 at 6q27 ( P =1.1 × 10 −8 , OR=1.08, logistic regression), lies 17 kb downstream of MIR3939 , which codes for microRNA 3939. Despite its proximity to MIR3939 , rs4710154 is an eQTL for RNASET2 in 11 tissues, including sun-exposed skin ( P =4.7 × 10 −19 , GTEx V6 analysis) and non-sun-exposed skin ( P =1.1 × 10 −7 , GTEx V6 analysis) [11] . This SNP is linked to rs9355610 ( r 2 =0.89, D ′=0.99, Supplementary Table 19 ), associated with Grave’s disease and Hashimoto’s thyroiditis [40] ; rs9355610 is also an eQTL for RNASET2 in sun-exposed ( P =1.0 × 10 −1 , GTEx V6 analysis) and non-sun-exposed skin ( P =1.6 × 10 −8 , GTEx V6 analysis) [11] . RNASET2 encodes ribonuclease T2, an evolutionarily conserved, ubiquitous RNase that inhibits cell proliferation (via stimulation of immune cells) and mediates cellular stress responses [41] . Accordingly, this enzyme has tumour suppressor activity in many cancer lines, including melanoma [42] , and has demonstrated pro-apoptotic activity in keratinocytes [43] . Interestingly, two of the 14 novel susceptibility variants reside near or within long non-coding RNA genes. rs2776353 at 21q22.3 ( P= 2.0 × 10 −14 , OR=0.91, logistic regression) is located 10 kb upstream of LINC00111 , while rs2294214 ( P= 3.1 × 10 −8 , OR=1.07, logistic regression) lies within an intron of CASC15 (also known as LINC00340 ); both SNPs have predicted enhancer and promoter activity in keratinocytes. A recent study compared the expression of long non-coding RNAs in BCC samples to that of normal skin controls and found that CASC15 was overexpressed in BCC [44] . Overexpression of CASC15 has also been implicated in melanoma progression and metastasis [45] . Our analysis of independent BCC expression data confirmed significant upregulation of CASC15 in BCC, further implicating this gene in BCC development. In addition to confirming the previously reported association of five pigmentation loci with BCC, we identified a novel susceptibility locus—rs10810657 at 9p22.2 ( P =1.5 × 10 −17 , OR=0.90, logistic regression)—that may also influence pigmentation. rs10810657, located 14 kb upstream of BNC2 , reached genome-wide significance in the meta-analysis and is an eQTL for BNC2 in blood ( Table 2 ). This SNP is in LD with rs12350739 ( r 2 =0.87, D ′=0.99, Supplementary Table 20 ), associated with human skin pigmentation via regulation of BNC2 transcription in melanocytes, and rs62543565 ( r 2 =0.7, D ′=0.87), associated with the age-related development of facial pigmented spots [46] , [47] . rs10810657 is also linked to rs2153271 ( r 2 =0.9, D ′=0.99), which is intronic to BNC2 and associated with freckling [48] . BNC2 codes for basonuclin 2, a protein thought to function both as an mRNA-processing enzyme and a transcription factor [46] . It is expressed in melanocytes and, to a lesser extent, keratinocytes, with higher expression levels corresponding to darker skin pigmentation [46] . In summary, this two-stage meta-analysis represents the largest GWAS for BCC and identified 14 novel susceptibility loci with roles in telomere maintenance, immune regulation and tumour progression. Further investigation of these loci will improve our understanding of BCC pathogenesis and improve our ability to prevent these common tumours. Stage 1 study design and population 23andMe Inc. (Mountain View, CA), a genetics company, provided free access to anonymized genetic and phenotypic information for stage 1 of this GWAS. All information came from 23andMe research participants who provided informed consent to participate in research, in accord with 23andMe’s human subjects protocol (reviewed and approved by Ethical and Independent Review Services, an AAHRPP accredited IRB). 23andMe gathers genetic information by genotyping sample material provided by its research participants; phenotypic information is collected via research participant responses to online surveys. Inclusion and exclusion criteria are discussed below. Sample sizes for cases and controls were not predetermined as the intention was to maximize the number of subjects in both groups; hence, all subjects passing inclusion and exclusion criteria were included, which resulted in 12,945 BCC cases and 274,252 controls. Stage 1 genome-wide association analysis Association analysis for stage 1 was performed using logistic regression, assuming an additive model for allelic effects. The analysis was adjusted for age, sex and population stratification (using the first five principal components), generating the following model: The association test P -value was computed using a likelihood ratio test. Results for the X chromosome were computed similarly, with male genotypes coded as if they were homozygous diploid for the observed allele. Additionally, test statistics were adjusted for genomic control to correct for residual population stratification persisting after principal component analysis; the genomic control inflation factor was 1.085 (computed from the median P -value for results that passed quality control). Genome-wide association analysis generated a set of index SNPs. The index SNPs show information for the most-associated SNP in each associated region. We define regions of interest by identifying SNPs with P <10 −5 , then grouping these into intervals separated by gaps of at least 250 kb, and choosing the SNP with smallest P within each interval. Stage 1 genotyping and quality control Samples were genotyped on one of four genotyping platforms. The V1 and V2 platforms were variants of the Illumina HumanHap550+ BeadChip, including about 25,000 custom SNPs selected by 23andMe, with a total of about 560,000 SNPs. The V3 platform was based on the Illumina OmniExpress+ BeadChip, with custom content to improve the overlap with our V2 array, with a total of about 950,000 SNPs. The V4 platform in current use is a fully custom array, including a lower redundancy subset of V2 and V3 SNPs with additional coverage of lower-frequency coding variation, and about 570,000 SNPs. Samples that failed to reach 98.5% call rate were re-analysed. Individuals whose analyses failed repeatedly were re-contacted by 23andMe to provide additional samples, as is done for all 23andMe research participants. Individuals were only included if they had >97% European ancestry, as determined through an analysis of local ancestry [49] . Briefly, this analysis first partitions phased genomic data into short windows of about 100 SNPs. Within each window, a support vector machine is used to classify individual haplotypes into one of 31 reference populations. The support vector machine classifications are then fed into a hidden Markov model (HMM) that accounts for switch errors and incorrect assignments, and gives probabilities for each reference population in each window. Finally, simulated admixed individuals are used to recalibrate the HMM probabilities so that the reported assignments are consistent with the simulated admixture proportions. The reference population data are derived from public data sets (the Human Genome Diversity Project, HapMap and 1000 Genomes), as well as 23andMe research participants who have reported having four grandparents from the same country. A maximal set of unrelated individuals was chosen for each analysis using a segmental identity-by-descent (IBD) estimation algorithm [50] . Individuals were defined as related if they shared more than 700 cM IBD, including regions where the two individuals share either one or both genomic segments identical-by-descent. This level of relatedness (roughly 20% of the genome) corresponds approximately to the minimal expected sharing between first cousins in an outbred population. Participant genotype data were imputed against the March 2012 ‘v3’ release of 1000 Genomes reference haplotypes [51] . Data for each genotyping platform were phased and imputed separately. First, Beagle [52] (version 3.3.1) was used to phase batches of 8000–9000 individuals across chromosomal segments of no more than 10,000 genotyped SNPs, with overlaps of 200 SNPs. SNPs with Hardy-Weinberg equilibrium P <10 −20 , call rate<95%, or with large allele frequency discrepancies compared to European 1000 Genomes reference data were excluded. Frequency discrepancies were identified by computing a 2 × 2 table of allele counts for European 1000 Genomes samples and 2000 randomly sampled 23andMe research participants with European ancestry, and identifying SNPs with a chi-squared P <10 −15 . Each phased segment was imputed against all-ethnicity 1000 Genomes haplotypes (excluding monomorphic and singleton sites) using Minimac2 [53] , using 5 rounds and 200 states for parameter estimation. For the non-pseudoautosomal region of the X chromosome, males and females were phased together in segments, treating the males as already phased; the pseudoautosomal regions were phased separately. Males and females were then imputed together using minimac, as with the autosomes, treating males as homozygous pseudo-diploids for the non-pseudoautosomal region. For quality control of genotyped GWAS results, SNPs that were only genotyped on the ‘V1’ platform were flagged due to small sample size, and SNPs on chrM or chrY because many of these are not currently called reliably. Using trio data, SNPs that failed a test for parent-offspring transmission were also flagged; specifically, the child’s allele count was regressed against the mean parental allele count, and SNPs with fitted β <0.6 and P <10 −20 for a test of β <1 were flagged. SNPs with a Hardy-Weinberg P <10 −20 in Europeans, or a call rate of <90%, were also flagged. Genotyped SNPs were also tested for genotype date effects, and SNPs with P <10 −50 by analysis of variance of SNP genotypes against a factor dividing genotyping date into 20 roughly equal-sized buckets were flagged. For imputed GWAS results, SNPs with avg.rsq<0.5 or min.rsq<0.3 in any imputation batch were flagged, as well as SNPs that had strong evidence of an imputation batch effect. The batch effect test was an F test from an analysis of variance of the SNP dosages against a factor representing imputation batch; results with P <10 −50 were flagged. Prior to GWAS, the largest subset of the data passing these criteria was identified for each SNP, based on their original genotyping platform—either v2+v3+v4, v3+v4, v3, or v4 only—and association test results were computed for whatever was the largest passing set. As a result, there were no imputed results for SNPs that failed these filters. When choosing between imputed and genotyped GWAS results, if either the imputed test passed quality control, or a genotyped test was unavailable, the imputed result was reported; otherwise, the genotyped result was reported. For tests using imputed data, imputed dosages were used rather than best-guess genotypes. Across all results, logistic regression results that did not converge due to complete separation, identified by abs (effect)>10 or stderr>10 on the log odds scale, were flagged. Linear regression results for SNPs with MAF<0.1% were also flagged, since tests of low frequency variants can be sensitive to violations of the regression assumption of normally distributed residuals [20] , [54] , [55] . Stage 1 associations using nearest genotyped SNP To assess the effect of imputation, we analysed the association between the nearest genotyped SNP at each locus and BCC, and then compared this association to that from the original imputed SNP. The genotyped results are consistent with the imputed results albeit slightly less significant. Stage 1 subset analyses Subset analysis by age and gender was performed for the genome-wide significant index SNPs in stage 1. For age-based analysis, the stage 1 cohort was divided into four age intervals with similar effective sample sizes based on case and control sample counts. Association test results were then computed within each of these age intervals for the 28 SNPs. The interaction between genotype effect and age interval was also calculated. For all these association tests, we used the same covariates used in stage 1: age, sex and five principal components. Thus, association tests within a specific age interval were still adjusted for age as a continuous covariate. For gender analysis, we compared effect sizes estimated in men versus effect sizes estimated in women for the 28 SNPs. We also performed logistic regression separately in the male and female subsets, and calculated P -values from a likelihood ratio test for adding a gender by genotype interaction to the full logistic regression models. For melanoma subset analysis, association tests for BCC were computed separately in melanoma controls and melanoma cases. Stage 1 phenotype categorization 23andMe identified BCC cases by using research participants’ self-reported answers to online questionnaires. Subjects who answered ‘Yes’ and/or selected BCC from a dropdown menu in response to at least one of the following questions were defined as cases: ‘Have you ever been diagnosed by a doctor with basal cell carcinoma?’, ‘What type of skin cancer did you have? Please check all that apply.’, ‘What type of skin cancer or cancers have you been diagnosed with? Please check all that apply.’ ‘Have you ever been diagnosed with basal cell carcinoma?’ ‘Have you ever been diagnosed or treated for any of the following conditions?’ Controls were defined as subjects who answered ‘No’ and did not select BCC from any relevant dropdown menus. In addition, subjects who answered ‘No’ to at least one of the following questions (and ‘Yes’ to none) were defined as controls: ‘Have you ever been diagnosed with cancer, including skin cancer or cancerous moles?’, ‘Has a doctor ever told you that you have a type of cancer?’, ‘Have you ever been diagnosed or treated with any of the following conditions?’ Among the samples with imputed genotypes, 23andMe has 12,945 BCC cases and 274,252 controls. Sensitivity and specificity of stage 1 self-reported data To assess the validity of self-reported phenotypic data in stage 1, 23andMe surveys (pertaining to skin cancer history and pigmentation) were randomly administered to patients seen in Stanford outpatient clinics. The survey answers were then compared to medical records to assess for accuracy with respect to BCC diagnosis to determine the sensitivity and specificity of the survey responses. P -values were determined using chi-square analysis. This sub-study was approved by the Stanford University Institutional Review Board with a waiver of documentation of informed consent. Stage 2 study design and population The Nurses’ Health Study was established in 1976, when 121 700 female registered nurses between the ages of 30 and 55 years residing in 11 larger US states completed and returned an initial self-administered questionnaire on their medical histories and baseline health-related exposures. Biennial questionnaires with collection of exposure information on risk factors have been collected prospectively. Every 2 years, along with exposures, outcome data with appropriate follow-up of reported disease events are collected. Overall, follow-up has been high; after more than 20 years, ∼ 90% of participants continue to complete questionnaires. From May 1989 through September 1990, we collected blood samples from 32,826 participants in the NHS. Information on BCC development was first collected in the 1984 questionnaire. The Health Professionals Follow-up Study (HPFS) was established in 1986 when 51,529 men from all 50 US states in health professions (dentists, pharmacists, optometrists, osteopath physicians, podiatrists and veterinarians) aged 40–75 years answered a detailed mailed questionnaire. The average follow-up rate for this cohort over 10 years is >90%. On each biennial questionnaire, we obtained disease- and health-related information. Between 1993 and 1994, 18,159 study participants provided blood samples by overnight courier. Information on BCC development was first collected in the 1986 questionnaire. The protocol for this study was approved by the Institutional Review Board at Brigham and Women’s Hospital and the Harvard School of Public Health. All of the participants provided informed consent. As in stage 1, all subjects passing inclusion and exclusion criteria were included, resulting in 4,242 BCC cases and 12,802 controls; sample sizes were not predetermined. Stage 2 genotyping and quality control There were 18 GWAS data sets from the NHS and HPFS as nested case-control studies with cleaned genotype data available. We combined these data sets into three complied data sets based on their genotype platform type: Affymetrix, Illumina HumanHap series or Illumina Omni Express. The Affymetrix data set was comprised of data on the Affy 6.0 platform (NHS-type 2 diabetes, NHS-coronary heart disease, HPFS-type 2 diabetes, HPFS-coronary heart disease). The Illumia HumanHap data set was comprised of several platforms: Illumina 550K (NHS-breast cancer, NHS-Pancreas cancer, HPFS-pancreas cancer), Illumina 610Q (NHS-kidney stone, HPFS-kidney stone, HPFS-prostate cancer) and Illumina 660 (NHS-glaucoma, HPFS-glaucoma). The Illumina Omni Express data set contained only studies genotyped on the Omni Express platform (NHS-endometrial cancer, NHS-colon cancer, NHS-mammographic density, NHS-gout, HPFS-colon, HPFS-gout). We combined the individual data sets that were genotyped on the same platform, removing any SNPs that were not in all studies and with a missing call rate>5%, and flipping strands where appropriate to create a final compiled data set. This resulted in 668,283 SNPs in the Affymetrix data set, 459,999 SNPs in the Illumina HumanHap data set and 565,810 SNPs in the Illumina Omni Express data set. Analyses were restricted to subjects with self-reported European ancestry. Genetic principal components were calculated using sets of independent SNPs (12,000–33,000 SNPs depending on platform). Subjects who did not cluster with other self-identified Europeans based on the top five principal components were also excluded. We then ran a pairwise IBD analysis for each combined data set to detect duplicate and related individuals based on resulting Z scores. If 0 ⩽ Z 0 ⩽ 0.1 and 0 ⩽ Z 1 ⩽ 0.1 and 0.9 ⩽ Z 2 ⩽ 1.1 then a pair was flagged as being identical twins or duplicates. Pairs were considered full siblings if 0.17 ⩽ Z 0 ⩽ 0.33 and 0.4 ⩽ Z 1 ⩽ 0.6 and 0.17 ⩽ Z 2 ⩽ 0.33. Half siblings or avunculars were defined as having 0.4 ⩽ Z 1 ⩽ 0.6 and 0 ⩽ Z 2 ⩽ 0.1. Some of the duplicates flagged in this step were expected, having been genotyped in multiple data sets and hence having the same cohort IDs. In this case, one of each pair was randomly chosen for removal from the data set. Instances where pairs were flagged as unexpected duplicates with the different cohort IDs, but pairwise genotype concordance rate>0.999, resulted in removal of both individuals from the pair. Related individuals (full sibs, half sibs/avunculars) were not removed from the final data sets. In the Affymetrix data set, 167 individuals were removed because they were duplicates or were flagged for removal from secondary genotype data cleaning, leaving a total of 8065 individuals. Of the 6894 individuals originally in the Illumina data set, 107 were removed because they were duplicates or flagged for removal in the genotyping step, leaving 6787 IDs. In addition, eight pairs of individuals were flagged as related. In the Omni express data set, there were 5956 individuals at the start, with 39 IDs to remove leaving 5917 IDs and 5 pairs of related IDs. After removing duplicate IDs and flagging related pairs of IDs, we used eigenstrat to run PCA analysis on each compiled data set, removing one member from each flagged pair of related individuals. For Affymetrix and Illumina HumanHap, we used approximately 12,000 SNPs that were filtered to ensure low pairwise LD [56] . For the OmniExpress data set we used approximately 33,000 SNPs that were similarly filtered. We plotted the top eigenvectors using R and examined the plots for outliers. Finally as a quality control check, we ran logistic regression analyses using each individual study’s controls as ‘cases’ and the rest of the studies controls as ‘controls’. For example, in the Illumina Omni Express data set, we ran regressions of NHS-gout controls considered as ‘cases’ versus the HPFS-gout, NHS-endometrial cancer, NHS-colon cancer, NHS-mammographic density and HPFS-colon cancer. We then ran regressions with each of the other study controls as ‘cases’ versus all of the rest of the controls. We looked for P values of genome-wide significance ( P <10 −8 ) and examined QQ plots to determine if any SNPs were flagged as significant where no SNPs should have been significant. In the Affymetrix data set 100 SNPs were flagged and removed. In the Illumina HumanHap data set, eight SNPs had P <10 −8 in any of the QC regressions and were removed. No SNPs in the Illumina Omni Express data set had P -values<10 −8 hence no additional SNPs needed to be removed. After the data sets were combined and appropriate SNP and ID filters applied, the complied data sets were imputed. Using combined GWAS genotypes on each genotyping platform and the 1000 Genomes Project ALL Phase I Integrated Release Version 3 Haplotypes excluding monomorphic and singleton sites (2010-11 data freeze, 2012-03-14 haplotypes) as reference panel, we imputed the genotypes of markers in the 1000 Genomes Project for 8065 samples in Affymetrix data set, 6787 samples in Illumina HumanHap data set and 5917 samples in Illumina Omni Express data set. SNP genotypes were imputed in three steps. First, genotypes on each chromosome were split into chunks to facilitate windowed imputation in parallel using ChunkChromosome (v.2011-08-05) ( http://genome.sph.umich.edu/wiki/ChunkChromosome ). Then each chunk of chromosome was phased using MACH (v.1.0.18.c) ( http://www.sph.umich.edu/csg/abecasis/MaCH/index.html ). In the final step, Minimac (v.2012-08-15) ( http://genome.sph.umich.edu/wiki/Minimac ) was used to impute the phased genotypes to approximately 31 million markers in the 1000 Genomes Project [51] . Sensitivity analysis in stage 2 Sensitivity analysis for five SNPs— IRF4 rs12203592, KRT5 rs11170164, PLIN3 rs10425559, NEU1 rs9267650 and EXOC2 rs12210050—using high imputation quality subsets was performed. Concordance for two SNPs (rs12916300 and rs35407) was compared between stage 2 imputed data and directly genotyped data among the overlapping samples of 251 controls and 280 cases. Direct genotyping was also performed for rs9275642 and rs1050529 in a subset of BCC cases and controls within NHS. The total sample size is 1204 with 661 cases and 543 controls. Stage 2 phenotype categorization Participants in both NHS and HPFS cohorts reported new BCC diagnosis biennially. Eligible cases in the NHS and HPFS consisted of participants with self-reported BCC any time after baseline up to the 2012 follow-up cycle for both cohorts. Samples free of BCC were controls in this study. In the three compiled data sets, samples without information on BCC diagnosis were excluded. Furthermore, all BCC cases with melanoma were also excluded. Among the samples with imputed genotypes, we have 1777 BCC cases and 5411 controls in Affymetrix data set, 1268 BCC cases and 3685 controls in Illumina HumanHap data set and 1197 BCC cases and 3706 controls in Illumina Omni Express data set totalling 4242 BCC cases and 12,802 controls. Validity of stage 2 self-reported data The identification of BCC cases in stage 2 was based on self-report without pathological confirmation. Because the participants in the cohorts were nurses and other health professionals, the validity of their reports was expected to be high and has been proven in validation studies: >90% confirmed by histopathology records [57] , [58] , [59] . In addition, previous studies of BCC in the NHS using self-reported cases identified both constitutional and sun-exposure risk factors as expected, such as lighter pigmentation, less childhood and adolescent tanning tendency, higher tendency to sunburn, and tanning salon attendance [58] , [60] . Moreover, in our previous study of BCC using the same cohorts as this study (NHS and HPFS), we confirmed the MC1R gene (a well-established pigmentation gene) as the most promising locus of BCC risk [4] . In addition, we identified many other pigmentation SNPs (for example, rs12203592 at IRF4 , rs1408799 at TYRP1 and rs12913832 at HERC2 ) in our data set with significant associations with BCC [4] . These genetic and non-genetic data together suggest that the bias due to self-report of BCC is likely to be minimal in our study. Stage 2 genome-wide association analysis We used ProbABEL software to test the GWAS association between minor allele counts and BCC risk using imputed dosage data. We performed logistic regression analysis under an additive model with adjustment for age, sex, BCC history and the first five principal components, generating the following model: These principal components were calculated for all individuals on the basis of approximately 10,000 unlinked markers using the EIGENSTRAT software [61] . Associations in each component GWAS set (Affymetrix, Illumina HumanHap series and Illumina Omni Express) were combined in an inverse-variance-weighted meta-analysis using the METAL software. Phenotype and environmental factors The amount of UV exposure based on residence location in 1986 was coded as a continuous variable. Information on pigmentation traits was collected from prospective questionnaires in both the NHS and HPFS using similar wording. We regressed ordinal coding for natural hair colour (1—red, 2—blonde, 3—light brown, 4—dark brown or black), tanning ability during adolescence (1—tans without burning (none/some redness only), 2—burns then tans, 3—burns/peels (painful burn with blisters)) and number of blistering sunburns (1=never, 2=1-2 times, 3=3–5 times, 4=6 times and above). Statistical models for pigmentation and UV exposure To clarify the influence of pigmentation traits on our associations, we additionally adjusted for these traits (hair colour, tanning ability during adolescence and number of blistering sunburns) in individual studies with ProbABEL. Associations in each component GWAS set (Affymetrix, Illumina HumanHap series and Illumina Omni Express) were combined in the same meta-analysis using the METAL software. The primary gene-risk factor interaction analytic model included each SNP and risk factor (UV exposure or pigmentation traits) and an SNP × risk factor interaction term, as well as age, sex and the first five principal components as covariates: The logistic regression analyses within each platform were conducted with ProbABEL. Associations in each component GWAS set (Affymetrix, Illumina HumanHap series and Illumina Omni Express) were combined in an inverse-variance-weighted meta-analysis using the METAL software. Meta-analysis For each SNP, meta-analysis was conducted to combine stage 1 and stage 2 results. Heterogeneity of per-SNP effect sizes in studies contributing to stage 1, stage 2 and the overall meta-analysis was assessed and fixed effects meta-analysis was conducted. The same method as in stage 1 was used to generate a set of index SNPs within each associated region. Top SNPs with P <5 × 10 −8 were finally reported. All R 2 and D ' between individual SNPs were calculated based on the 1000 Genomes Pilot 1 data set, CEU Population ( http://www.broadinstitute.org/mpg/snap/ldsearchpw.php ) [62] . Proportion of familial relative risk We have used the formula for calculating the proportion of FRR as outlined by the Cancer Oncological Gene-environment Study ( http://www.nature.com/icogs/primer/common-variation-and-heritability-estimates-for-breast-ovarian-and-prostate-cancers/#70 ) as described previously [63] . The odds ratios derived from our meta-analysis of stages 1 and 2 are assumed to be relative risks. We estimated the proportion of the FRR explained by each SNP (FRR snp ) as: Here, the risk allele and alternative allele frequencies are p and q , respectively, and r is the odds ratio for the risk allele. Allele frequencies derived from the 1000 Genomes Project European population data. Assuming that the loci combine multiplicatively and are not in LD, the combined effect of all loci is given by: Here, the product is across all loci. The proportion of the familial relative risk attributable to the SNPs, on a log scale, is then given by: In this equation, λ P is the familial relative risk observed in epidemiological studies. λ P is 2.6-fold for BCC [60] , [64] . Regulatory function of novel variants For each novel BCC susceptibility variant, we searched for evidence of regulatory function using recently updated HaploReg version 4 ( http://www.broadinstitute.org/mammals/haploreg/haploreg.php ) [65] , [66] . We queried each rsID and extracted data from ENCODE Project Consortium 2011–2012 on closest annotated gene, ChIP-Seq transcription factor binding, DNaseI hypersensitivity sites, and enhancer and promoter chromatin segmentation states [67] , [68] , [69] . We also extracted data from Roadmap Epigenomics Consortium 2015 on enhancer and promoter chromatin segmentation states, specifically using the following states: 15-state HMM, 25-state HMM, H3K4me1, H3K4me3, H3K27ac and H3K9ac [70] . We particularly focused on enhancer and promoter annotations that referenced normal human epidermal keratinocytes (NHEK) and primary foreskin keratinocytes. Finally, we used HaploReg v4 to extract eQTL data for each variant, as version 4 is updated with cis eQTL data from the GTEx pilot analysis and other studies [11] . We made special note of variants that were eQTLs in skin tissue. Gene expression analysis Processed gene-expression data for BCC and normal skin (GSE53462 and GSE7553) were obtained from the GEO ( http://www.ncbi.nlm.nih.gov/geo/ ) [71] , [72] , [73] . Fifteen BCC samples and five controls were included for GSE7553; for GSE53462, nine ‘classic-type’ BCC samples were included, along with five controls. Each gene of interest was selected by its proximity to one of the 14 novel risk variants; however, if a variant was an eQTL in skin tissue for a more distant gene, then this gene was chosen instead. For each data set, Geo2R, which employs a linear-based model for microarray analysis, was utilized to compare gene expression between BCC and normal skin controls [74] . Significant results were defined as instances of differential gene expression (in BCC tissue relative to control) reaching P <0.05 in both data sets. Regional association and forest plots Regional plots of –log10 ( P values) were generated using Locus Zoom [75] . Where pairwise LD measures are given, using LD data from the March 2012 release of 1000 Genomes data. To preserve detail, results with P <10 −100 are set to 10 −100 . In the plots, an ‘o’ symbol indicates a genotyped SNP and a ‘+’ indicates an imputed SNP. Colour indicates strength of LD with the index SNP. Forest plots were generated using the R forest plot package ( https://cran.r-project.org/web/packages/forestplot/forestplot.pdf ) [76] . Power calculations Power was computed according to Freidlin et al. [77] . To account for misclassification, expected genotype frequencies in study cases were replaced with a mixture of genotype frequencies in true cases and in true controls. Power was plotted as a function of odds ratio for detecting a variant with minor allele frequency 0.1, based on the GWAS sample size and with hypothetical misclassification rates of 0, 10 and 20% (where the specified fraction of study cases are misclassified controls). Data availability GWAS data from 23andMe and Nurses ‘Health/Health Professionals’ Study have not been deposited in public repositories, as consent for this was not obtained in the study protocols. The pre-computed rankings and P -values for SNPs included in the stage 1 GWAS are available upon request by contacting D.A.H. at dhinds@23andMe.com . Pre-computed rankings and P -values for the top 10,000 SNPs included in the stage 2 GWAS are freely available by contacting www.channing.harvard.edu/nhs . Processed gene-expression data for BCC and normal skin are freely available from GEO ( http://www.ncbi.nlm.nih.gov/geo/ ) using the accession numbers GSE53462 (ref. 72 ) and GSE7553 (ref. 73 ). Any additional data (beyond those included in the main text and Supplementary Information ) that support the findings of this study are available from the corresponding author upon request. How to cite this article: Chahal, H. S. et al. Genome-wide association study identifies 14 novel risk alleles associated with basal cell carcinoma. Nat. Commun. 7:12510 doi: 10.1038/ncomms12510 (2016).